Modular assembly of optical nanocircuits A key element enabling the microelectronic technology advances of the past decades has been the conceptualization of complex circuits with versatile functionalities as being composed of the proper combination of basic ‘lumped’ circuit elements (for example, inductors and capacitors). In contrast, modern nanophotonic systems are still far from a similar level of sophistication, partially because of the lack of modularization of their response in terms of basic building blocks. Here we demonstrate the design, assembly and characterization of relatively complex photonic nanocircuits by accurately positioning a number of metallic and dielectric nanoparticles acting as modular lumped elements. The nanoparticle clusters produce the desired spectral response described by simple circuit rules and are shown to be dynamically reconfigurable by modifying the direction or polarization of impinging signals. Our work represents an important step towards extending the powerful modular design tools of electronic circuits into nanophotonic systems. The lumped element model in electronics is a simplified description of a spatially distributed physical system based on a topology consisting of discrete entities. This well-established approximation is justified by the small dimensions of the circuit elements compared with the operating wavelength. Small colloidal metallic and dielectric nanoparticles (NPs), readily synthesized with conventional chemical processes, are the ideal platforms to translate these concepts to optical frequencies. Using optical nanocircuit concepts [1] , [2] , [3] , [4] , the intrinsic optical impedance of NPs may be controlled by their geometry and material composition. This impedance is defined as the ratio of the local potential difference V = |E| l and the flux of displacement current I d =− iω | E| S through the NP [1] , [2] , [3] , [4] , where E is the local electric field vector, l is the NP length along the electric field, ω is the frequency of operation, ε is the NP dielectric constant and S is its transverse cross-section. It follows that a dielectric NP with Re( ε ) >0 behaves as a nanocapacitor, while a metallic NP with Re( ε ) <0 acts as a nanoinductor. Ohmic loss in the materials takes the role of a nanoresistor. When retardation can be neglected, these quantities are shown to satisfy Kirchhoff’s circuit laws [1] . It is therefore tantalizing to translate the electronic circuit concepts to optical frequencies. Modularizing the optical response of NPs and treating them as lumped elements that can be connected into complex circuits is at the basis of the ‘metatronic’ paradigm. Metatronic concepts have provided a useful theoretical framework connecting plasmonics, metamaterials and nanophotonics with conventional electronics [2] , [3] , [4] , [5] . These ideas have guided the efficient design of metasurfaces [6] , [7] and the modelling of a variety of composite nanostructures, including plasmonic NP clusters [8] , [9] , [10] , NP rings exhibiting strong optical magnetism [11] and microcavity lasers [12] . However, the direct application of these concepts to photonic circuits has so far been limited to modelling and tuning optical nanoantennas [13] , [14] , [15] , [16] , [17] , [18] , [19] , and to realizing a ladder network of two-dimensional (2D) nanoinductors and nanocapacitors in the form of a subwavelength grating at mid-infrared frequencies [4] . These earlier experiments have demonstrated nanocircuits with limited complexity and specific symmetry constraints. Most importantly, no prior experiment has been able to show the modular use of optical circuit elements, dynamically connected in different ways to realize complex circuit topologies of choice. In this paper, we introduce new theoretical concepts and improved nanomanipulation techniques to experimentally verify the full potential of the photonic circuit concepts, allowing for the design, assembly and interrogation of relatively complex optical nanocircuit topologies. After identifying NPs with the desired optical impedance, we dynamically assemble them into nanocircuits using atomic force microscope (AFM) nanomanipulation. The flexibility of this assembly approach enables arrangement of NPs into chosen geometries, determined by circuit rules, to synthesize the desired spectral response in photonic circuits of increasing complexity. By comparing our far-field optical scattering measurements with full-wave simulations and a suitably developed circuit model, we prove that the assembled NP clusters indeed operate as complex optical nanofilters with a rather intuitive circuit topology. While it is known that anisotropic photonic nanostructures can exhibit strong polarization-controlled response [20] , [21] , here we exploit this concept to demonstrate ‘stereocircuits’. These stereocircuits are reconfigurable by changing the direction and/or polarization of the incident light, a possibility not available in conventional electronic circuits. Assembly and characterization of NP clusters In our experiments, we initially dispersed a mixture of gold NPs (~60 nm in diameter) and Al 2 O 3 NPs (~45 nm in diameter) on a glass substrate. The AFM image of the sample ( Fig. 1a ) allowed us to locate each NP but did not distinguish between different NP types without ambiguity. To solve this issue, we mapped the same area using optical dark-field microscopy (see Methods section for details), from which only scattering signals from Au NPs were detectable ( Fig. 1b ). Correlating the AFM and optical scattering images allowed us to differentiate metallic NPs (nanoinductors) from dielectric NPs (nanocapacitors) with certainty. By measuring the scattering from each NP, we detected differences in the scattering spectra because of slight variations in NP shape and size. Similar to the actual circuit design process, we then picked a few chosen NPs with the desired impedance and assembled them to produce series, parallel and more complex connections ( Fig. 1c ) using the AFM tip. Finally, dark-field scattering measurements, shown schematically in Fig. 1d , were used to confirm the functionality of the nanoclusters by comparing the measured scattering spectra with the predicted nanocircuit response. 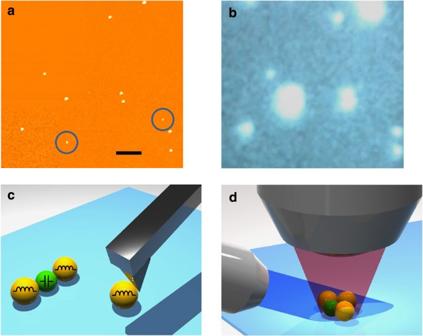Figure 1: Assembly and characterization of a modular optical nanocircuit. (a) AFM and (b) dark-field scattering images of plasmonic and dielectric NPs randomly distributed on a glass substrate. Only Au NPs yield strong scattering signals. Scale bar, 3 μm. The NPs enclosed in circles inaare missing inb, thereby identifying them as dielectric NPs. (c) Illustration of AFM nanomanipulation as a way to dynamically assemble complex optical nanocircuits from independent optical inductors (plasmonic NPs, yellow) and capacitors (dielectric NPs, green). (d) Schematic representation of our dark-field scattering measurements. Light impinges at an incidence angle of 60 degrees and the scattering signal is collected along the substrate normal (see Methods for details). Figure 1: Assembly and characterization of a modular optical nanocircuit. ( a ) AFM and ( b ) dark-field scattering images of plasmonic and dielectric NPs randomly distributed on a glass substrate. Only Au NPs yield strong scattering signals. Scale bar, 3 μm. The NPs enclosed in circles in a are missing in b , thereby identifying them as dielectric NPs. ( c ) Illustration of AFM nanomanipulation as a way to dynamically assemble complex optical nanocircuits from independent optical inductors (plasmonic NPs, yellow) and capacitors (dielectric NPs, green). ( d ) Schematic representation of our dark-field scattering measurements. Light impinges at an incidence angle of 60 degrees and the scattering signal is collected along the substrate normal (see Methods for details). Full size image A basic LC optical nanocircuit We start from the most basic nanocircuit consisting of a single Au nanosphere with radius a ≅ 30 nm excited by a uniform electric field, as shown schematically in Fig. 2a with its AFM image as inset. Its corresponding scattering measurement is reported in Fig. 2b , showing a clear resonant peak around λ 0 =550 nm. This measurement can be accurately predicted and explained with the nanocircuit model shown in Fig. 2c . 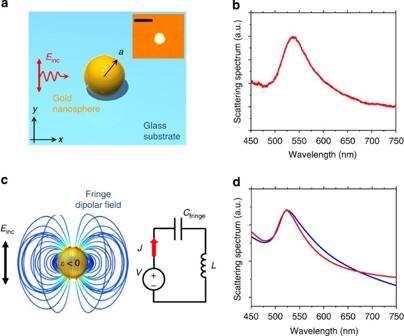Figure 2: An optical nanoinductor realizing a lumped LC circuit. (a) AFM image and illustration of a single Au NP on a glass substrate. Scale bar, 100 nm. (b) Dark-field scattering measurement. (c) Simulated fringe dipolar field lines (3D view) around the nanosphere when Re[ε] <0 and corresponding Thevenin-equivalent nanocircuit model. (d) Comparison between the scattering spectrum calculated with full-wave numerical simulations (red line) and the response predicted by nanocircuit theory (blue line; amplitude of the currentJflowing in the circuit inc, properly scaled for comparison). A single metallic nanosphere (Re[ ε ]<0) in this circuit representation is simply an inductor with optical impedance [1] Figure 2: An optical nanoinductor realizing a lumped LC circuit. ( a ) AFM image and illustration of a single Au NP on a glass substrate. Scale bar, 100 nm. ( b ) Dark-field scattering measurement. ( c ) Simulated fringe dipolar field lines (3D view) around the nanosphere when Re[ ε ] <0 and corresponding Thevenin-equivalent nanocircuit model. ( d ) Comparison between the scattering spectrum calculated with full-wave numerical simulations (red line) and the response predicted by nanocircuit theory (blue line; amplitude of the current J flowing in the circuit in c , properly scaled for comparison). Full size image connected in series with a capacitor of impedance Z fringe =(− iωε 0 2 πa ) −1 associated with the fringing fields around the sphere [1] ( ε 0 is the background permittivity). The optical circuit is driven by a voltage generator associated with the applied fields. The geometry and material properties of this particular nanosphere yield a small nanoinductance L ≅ 18.56 femtoH and fringe nanocapacitance C f ≅ 1.67 attoF, at λ 0 =550 nm. It should be noted that the proposed circuit model is different from the one originally formulated in ref. 1 and considered in previous papers on the topic. As detailed in the Methods section, the introduction of this alternative circuit model, which consists of the Thevenin equivalent of the circuit used in ref. 1 , is necessary here to properly relate the measured scattering spectra to a circuit quantity. The scattered fields are sustained by the polarization currents induced in the NPs. The polarization currents are directly related to the (displacement) current flowing into the circuit, indicated by the red arrow in Fig. 2c , when driven by a Thevenin voltage generator (see Methods). The frequency dependence of the current amplitude (blue curve in Fig. 2d ) agrees well with the scattering signals obtained experimentally ( Fig. 2b ) and calculated from full-wave simulations (red curve in Fig. 2d ). It is evident that the proposed nanocircuit model, despite its simplicity, captures not only the resonance frequency but also the frequency dispersion and resonance quality factor of the measured spectra. Adding complexity with higher-order nanocircuits Next, we consider a three-particle nanocircuit consisting of a dielectric Al 2 O 3 NP sandwiched between two Au NPs, as shown in Fig. 3a . Plotted in Fig. 3b are the measured scattering spectra from this nanocluster using s -polarized light, with the incident electric field either perpendicular to the NP array ( Y -circuit, blue line) or along it ( X -circuit, red line). Owing to the anisotropy of this nanocluster, the optical response exhibits a spectral shift dependent on the direction of the impinging field relative to the NP array. A red shift in resonant wavelength is expected for the X -circuit because of increased capacitive coupling among NPs, and it is reflected both in our experiments ( Fig. 3b ) and full-wave simulations ( Fig. 3c ). 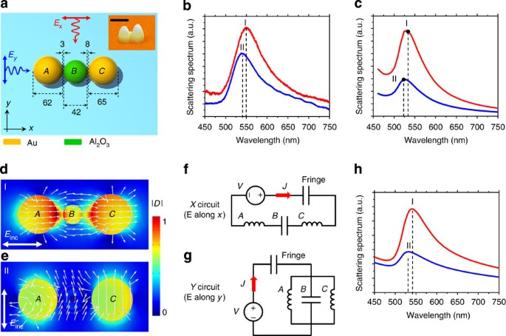Figure 3: Second and third order lumped nanofilters. (a) AFM image and geometry of a 3-NP cluster composed of an Al2O3NP sandwiched between two Au NPs. All dimensions are in nanometres. Scale bar, 100 nm. (b) Dark-field scattering measurements fors-polarized light exciting the nanocircuit with the electric field alongx(red line) ory(blue). Experimentally, the sample was rotated to allow light incident from different sides of the NP cluster. (c) Corresponding full-wave simulations with electric field alongx(red line) ory(blue). (d,e) Simulated electric displacement field distributions and field vectors at the resonance wavelengths for the two incidence directions:λ=532 nm (d, I) andλ=524 nm (e, II), as indicated by the vertical dashed lines and roman numbers inc. (f,g) Thevenin nanocircuit models of second order (f,X-circuit, series LC) and third order (g,Y-circuit, CLC) lumped nanofilters. The calculated fringe capacitance isCf≅18.79 attoF for theX-circuit configuration andCf≅3.75 attoF for theY-circuit. The impedance of the other elements can be calculated using Equation (1) and is independent of the circuit configuration. (h) Corresponding circuit theory predictions:X-circuit (red line) andY-circuit (blue). Figure 3d,e shows the corresponding simulated displacement vector distributions at the two resonant wavelengths: λ =532 nm for incident electric field parallel to the x axis ( Fig. 3d ; point I in Fig. 3c ) and λ =524 nm for electric field along the y axis ( Fig. 3e ; point II in Fig. 3c ). Similar to a conventional electronic circuit, the intrinsic nanoinductance of the gold NPs is not affected by other components in the circuit, despite their close proximity, and its value remains the same. Equation (1) also provides the nanocapacitance C ≅ 2.61 attoF for the Al 2 O 3 sphere, which is also independent of the surrounding. The associated fringe capacitance, instead, is slightly affected by the new circuit configuration because of the different fringe field distribution, as detailed in the caption of Fig. 3 and in the Methods section. Figure 3: Second and third order lumped nanofilters. ( a ) AFM image and geometry of a 3-NP cluster composed of an Al 2 O 3 NP sandwiched between two Au NPs. All dimensions are in nanometres. Scale bar, 100 nm. ( b ) Dark-field scattering measurements for s -polarized light exciting the nanocircuit with the electric field along x (red line) or y (blue). Experimentally, the sample was rotated to allow light incident from different sides of the NP cluster. ( c ) Corresponding full-wave simulations with electric field along x (red line) or y (blue). ( d , e ) Simulated electric displacement field distributions and field vectors at the resonance wavelengths for the two incidence directions: λ =532 nm ( d , I) and λ =524 nm ( e , II), as indicated by the vertical dashed lines and roman numbers in c . ( f , g ) Thevenin nanocircuit models of second order ( f , X- circuit, series LC) and third order ( g , Y- circuit, CLC) lumped nanofilters. The calculated fringe capacitance is C f ≅ 18.79 attoF for the X- circuit configuration and C f ≅ 3.75 attoF for the Y- circuit. The impedance of the other elements can be calculated using Equation (1) and is independent of the circuit configuration. ( h ) Corresponding circuit theory predictions: X -circuit (red line) and Y -circuit (blue). Full size image On the basis of the different electric displacement field distributions ( Fig. 3d,e ), two circuits with different connections among the elements ( Fig. 3f,g ) account for the change in the scattering spectra. The three nanocircuit elements are connected in series ( X -circuit in Fig. 3f ) for incident electric field polarized along the axis of the NP cluster, since this excitation ensures the continuity of the displacement current across the cluster, as confirmed by our simulations in Fig. 3d . In conventional circuit theory, the order of a filter is determined by the number of independent reactive elements. Accordingly, the X -circuit ( Fig. 3f ) realizes a second order filter, which is an LC circuit formed by the series combination of an inductor (the Au NPs) and a capacitor (determined by the Al 2 O 3 NP and the fringing fields). Conversely, for incident electric field perpendicular to the axis of the NP cluster ( Fig. 3e ), each element experiences the same potential difference (that is, voltage), leading to a parallel connection between them. This Y -circuit ( Fig. 3g ) forms a third order nanofilter, in which the fringe capacitance is connected in series to the parallel of the Au NP inductors and the Al 2 O 3 NP capacitor. The scattering spectra predicted by our circuit model ( Fig. 3h ) are indeed quantitatively consistent with the measured and simulated spectra for both X - and Y -circuits ( Fig. 3b,c ). By realizing different circuit configurations controlled by the direction of the excitation field, we are able to experimentally prove the design and operation of optical stereocircuits, which do not have a counterpart in the electronic realm. Thanks to this feature, we are able to encode different optical circuit responses within the same nanocluster, opening the possibility of parallel information processing and multiplexing at the nanoscale. Finally, we present an example of a circuit consisting of four NPs, which offers a richer response than the optical nanocircuits demonstrated in any previous experiment. Additional complexity and functionality are introduced by adding a metallic NP below the previous nanocircuit design, as illustrated in Fig. 4a . The scattering measurements shown in Fig. 4b were taken with incident light direction fixed while gradually changing the polarization from p to s . In both experiments ( Fig. 4b ) and full-wave simulations ( Fig. 4c ), two scattering resonances dominate the response: the first peak at longer wavelengths experiences a drastic boost going from p- to s polarization, while the second resonance at shorter wavelengths evolves from a sharper peak to a plateau-like response. Shown in Fig. 4d,e are the simulated displacement vector distributions at the longer wavelength resonance ( λ =688 nm), for polarizations parallel ( Fig. 4d ) and orthogonal ( Fig. 4e ) to the array, highlighting the polarization-dependent interaction among NPs. Even in this more complex configuration, the electric displacement vector distributions fully support the circuit models reported in Fig. 4f,g , which correspond to fourth order nanofilters. In the X -circuit ( Fig. 4f ), the additional nanoinductor (nanosphere D in Fig. 4a ) is in parallel with the nanocapacitor, as they share the same applied potential (see Fig. 4d ). In contrast, for the Y -circuit ( Fig. 4g ), the same nanoinductor is in series with the third order nanofilter analysed in Fig. 3 . This example shows that we can quantitatively control the spectral response by connecting an additional nanoinductor, in exactly the same way as in an electronic circuit. More specifically, we have been able to add a new zero and/or pole to the scattering response by adding an independent reactive element to the circuit of Fig. 3 . With similar principles, we may be able to design even more complex filtering functionalities by tailoring the position of such zeros and poles on the complex frequency plane, as routinely performed in electronic filter design [22] . As further discussed in Supplementary Note 1 and Supplementary Fig. 1 , the modular optical nanocircuits experimentally demonstrated here may indeed pave the way towards the realization of a wide range of filter responses based on lumped optical nanocircuit elements. We should emphasize that the nanocircuit paradigm unveiled by our experiments is significantly more powerful than equivalent circuit models for photonic structures previously developed [23] , [24] , [25] . Rather than modelling a distributed photonic system with an equivalent circuit, our work shows that it is actually possible to synthesize a photonic circuit functionality by assembling modular lumped nanoelements, providing a one-to-one correspondence between the desired circuit response and the topological design. 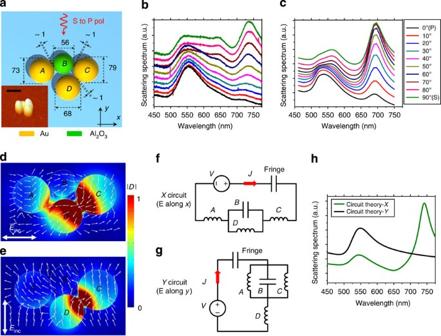Figure 4: A fourth order lumped nanofilter. (a) AFM image and geometry of a 4-NP complex nanocircuit composed of three Au NPs and one Al2O3NP. All dimensions are in nanometres (see Methods section andSupplementary Note 2for a thorough discussion on the effect of interparticle gaps). Scale bar, 100 nm. (b) Dark-field scattering measurements for polarization rotating fromstop; (c) corresponding full-wave simulations. Curves inb,chave been shifted vertically to facilitate comparisons. (d,e) Simulated electric displacement field distributions and field vectors for polarizations parallel (d) and orthogonal (e) to the array axis, at the longer wavelength resonance (λ=688 nm). (f,g) Thevenin nanocircuit models: the calculated fringe capacitance isCf≅7.72 attoF for theX-circuit (f) andCf≅5.62 attoF for theY-circuit (g). The impedance of the other elements can be calculated using Equation (1) and is independent of the circuit configuration. (h) Corresponding circuit theory predictions for the two orthogonal polarizations. Figure 4: A fourth order lumped nanofilter. ( a ) AFM image and geometry of a 4-NP complex nanocircuit composed of three Au NPs and one Al 2 O 3 NP. All dimensions are in nanometres (see Methods section and Supplementary Note 2 for a thorough discussion on the effect of interparticle gaps). Scale bar, 100 nm. ( b ) Dark-field scattering measurements for polarization rotating from s to p ; ( c ) corresponding full-wave simulations. Curves in b , c have been shifted vertically to facilitate comparisons. ( d , e ) Simulated electric displacement field distributions and field vectors for polarizations parallel ( d ) and orthogonal ( e ) to the array axis, at the longer wavelength resonance ( λ =688 nm). ( f , g ) Thevenin nanocircuit models: the calculated fringe capacitance is C f ≅ 7.72 attoF for the X- circuit ( f ) and C f ≅ 5.62 attoF for the Y- circuit ( g ). The impedance of the other elements can be calculated using Equation (1) and is independent of the circuit configuration. ( h ) Corresponding circuit theory predictions for the two orthogonal polarizations. Full size image The simple nanocircuit models that we have used to design this 4-NP cluster obviously cannot reproduce all the features captured by our full-wave simulations and experimental measurements. Nevertheless, our theory quantitatively predicts the changes in the measured response for the two orthogonal polarizations, as clearly shown in Fig. 4h . Namely, the scattering peak at shorter wavelengths becomes dominant (and the peak at longer wavelengths is suppressed) when the effective connection of the fourth metallic NP with the capacitor is changed from ‘in parallel’ to ‘in series’. For polarizations in between these two cases, the elements are neither in series nor in parallel. Instead, they are joined by ‘intermediate’ connections, unavailable in a conventional electronic circuit [26] , [27] . In this final section, we would like to emphasize the key message of our work: the nanocircuit paradigm provides an unmatched degree of simplicity to control and tailor the optical response of rather complex nanophotonic structures. Remarkably, the impedance of each nanosphere, which is directly calculated using Equation (1), remains independent of the cluster geometry and surrounding environment in all the circuits we have demonstrated, starting from the isolated NP to the complex fourth order nanocircuit (see Methods section for further details). In other words, each NP carries an inherent optical impedance, which is a property of the particle itself, allowing us to modularize its response and combine it in complex configurations. The distance between neighbouring NPs is expected to influence the overall response of the cluster; however, it does not directly affect the connection between NPs in the considered model. This is explained by the fact that we are considering here very small gaps between neighbouring particles. Under this condition, the flux of electric displacement vector is continuous from one particle to the next one, in the case of a series connection, or the electric field line integral across two neighbouring NPs is the same, in the case of a parallel connection. This ensures that the circuit elements may be truly considered to be connected in ‘series’ or ‘parallel’, while the different fringe field distribution can be simply modelled by a modified fringe capacitance (see Methods section). As the gaps grow, we need to consider the additional associated impedance, as described in refs 13 , 18 . The additional gap capacitances may result in noticeable spectral shifts, as expected and seen in Supplementary Fig. 2 (and corresponding Supplementary Note 2 ), but the overall nanocircuit response is preserved. As the interparticle distance grows even farther, even the notion of lumped element breaks down, and the coupling between particles needs to be modelled with nonlocal circuit elements, as discussed in ref. 28 . The very good agreement between our experimental results and theoretical predictions in the examples considered here demonstrates that for small gaps it is possible to neglect parasitic and nonlocal effects, resulting in these simple models. In summary, we have demonstrated the design and operation of several ‘stand-alone’ optical nanocircuits, without the geometry and symmetry constraints imposed in previous experiments on nanocircuits [4] , [18] . The modularization of the optical response by means of lumped optical elements has allowed us to design photonic nanocircuits of increasing complexity by connecting our basic building blocks, nanoinductors and nanocapacitors, in different topologies. In all the cases considered here, we have obtained remarkably good agreement between experiments, full-wave simulations and nanocircuit theory. For more sophisticated topologies, we envision the use of epsilon-near-zero background materials, which act as photonic insulators for the optical displacement current [3] and remove the undesired coupling between different nanocircuit elements because of displacement current ‘leakage’ (in Supplementary Note 1 we further discuss the primary limitations to scale up the complexity and ways to overcome them). While in these presented experiments we measured the nanocircuit response in the far-field, limited by diffraction, we envision that in a fully functional nanocircuit board, distributed nanoantennas [16] along the circuit will be able to interrogate and feed signals at the nanoscale, well below the limits dictated by diffraction. In light of these findings, the incorporation of NPs made of different materials in the same cluster, using top-down, bottom-up or hybrid fabrication approaches, may produce a variety of interesting prototypical nanocircuits with designed functionalities. Such nanocircuits may be integrated into nanophotonic systems for parallelized optical signal processing at the nanoscale. Sample preparation and AFM nanomanipulation Photolithographical marks were deposited on a glass coverslip to locate particular areas across its surface. The patterned substrate was then cleaned by 1–2% Hellmanex-II solution for 60 min in a sonication bath at ~30 °C temperature. Gold nanospheres (~60 nm in diameter, British Biocell EM.GC60) with 1 × 10 9 particles ml −1 were sonicated for 20 s and then deposited by a spin-coating procedure consisting of multiple speed steps (800, 2,000 and 4,000 r.p.m.). The details of the AFM nanomanipulation method can be found in refs 29 , 30 . The dimensions of the assembled NP clusters were experimentally determined with a limited accuracy (~a few nanometres). There are mainly two challenges in this operation: first, AFM images have a relatively poor resolution in the lateral directions, which is limited by the tip convolution effect. This challenge is particularly serious in our setup because we have chosen AFM tips with proper spring constant and large radius of curvature (~10 nm), so that the tip can be used to effectively manipulate NPs without breaking. The second challenge is related to the deviation of the NP shape from ideal spheres assumed in numerical simulations, as evident in the scanning electron microscopy image in Fig. 5a . In our effort to estimate the gap sizes, we take line cuts through the AFM images. We use the height of a NP as an estimate of its diameter and measure the centre-to-centre distance between NPs (that is, separation between intensity peaks in the AFM images). The gap size can be estimated by subtracting the NP size from the separation. As an example of the challenges of this operation, in the AFM images and line cuts shown in Fig. 5b–d , this approach actually leads to negative values of the apparent gap sizes, which is clearly not physical and likely due to the presence of facets or corners. Experimentally, we push the NPs as close as possible, knowing that the capping molecules on the surface of the NPs keep them from physically touching. 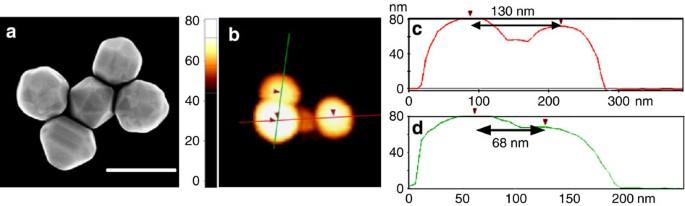Figure 5: Estimating the gap size between NPs. (a) Scanning electron microscopy image of a gold particle cluster on a conductive substrate, clearly showing facets and corners of the nanoparticles, leading to deviations from the ideal spherical shape. Scale bar, 200 nm (b) AFM image of the 4-nanoparticle nanocircuit presented inFig. 4. (c,d) Example of line cuts through the AFM image used for gap size estimation. Figure 5: Estimating the gap size between NPs. ( a ) Scanning electron microscopy image of a gold particle cluster on a conductive substrate, clearly showing facets and corners of the nanoparticles, leading to deviations from the ideal spherical shape. Scale bar, 200 nm ( b ) AFM image of the 4-nanoparticle nanocircuit presented in Fig. 4 . ( c , d ) Example of line cuts through the AFM image used for gap size estimation. Full size image Our simulations predict gap sizes on the order of nanometres, which corresponds to the uncertainty level encountered in experiments. In simulations, we started from reasonable dimensions extracted from the experiments and we then tuned the gap sizes by less than a few nanometres until we reached the best agreement between the experiments and theory. We have also verified that the characteristic scattering features of the nanocircuits are robustly preserved under small perturbations of the geometry, as further detailed in Supplementary Note 2 and Supplementary Fig. 2 . Dark-field scattering spectrum measurements Linear polarized white light excited the NP clusters as illustrated in Fig. 1d . The light was focused through a microscope objective with numerical aperture of 0.28 from an oblique incidence angle (that is, 60 degrees from the substrate normal). A long working distance objective with numerical aperture of 0.7 was used to collect the scattering signal along the substrate normal. The collected light was then focused on the entrance slit of an imaging spectrometer and detected with a nitrogen-cooled Si-CCD. When taking scattering spectra with impinging light from different directions relative to the assembled nanocluster, we rotated the sample mounted on both a rotational and a three-dimensional translation stage. We identified the same cluster by using the grid on the patterned substrate and patterns formed by nearby NPs. Circuit theory The impedance of all the circuit elements was calculated using Equation (1), with the actual dimension and material properties of the NPs. The values of permittivity as a function of frequency were taken from empirical data sets. The fringe field distribution, in the 3- and 4-NP clusters ( Figs 3 and 4 ), was modelled by a modified fringe capacitance. In order to estimate the modified fringe values, we considered the formula for a single particle, Z fringe =(− iωε 0 2 πa ) −1 , and we chose an optimized effective radius a, comparable to the dimension of the cluster in the direction of the incident electric field. This modelling is accurate as long as the distance between neighbouring particles is small, as explained in the Discussion section. We adopted here a modified circuit model compared with the one originally proposed in ref. 1 . In the case of the single NP shown in Fig. 2 , we used a series connection between the nanosphere impedance, the fringe capacitance and a voltage source related to the impinging wave, which is the equivalent Thevenin circuit of the one introduced in ref. 1 . This is motivated by the reasons discussed in the main text and in the following. Our experimental observations to determine the response of the nanocircuits are all carried out in the far-field region, for which the observable quantity of interest is the scattered energy measured by our dark-field microscope. Far-field scattering is directly related to the polarization currents induced on the NPs; therefore, in order to relate the measured far-field response to our optical nanocircuit model we need to ensure a direct relation between a quantity measurable in the circuit and the far-field scattering. In the seminal nanocircuit theory paper [1] , this issue was not a concern. It was shown that a subwavelength plasmonic NP illuminated by an incident wave can be modelled as an inductance, connected in parallel with a capacitance representing the fringe dipolar field, and driven by a current source, as shown in Fig. 6a . The continuity of the normal component of the displacement field with respect to the NP surface guarantees that the currents in the different branches of the equivalent circuit indeed obey Kirchhoff’s current law. Although this circuit model correctly predicts the resonance frequency of the plasmonic NP, it is difficultly related to far-field scattering measurements associated with the polarization current flowing along the circuit. At resonance, for instance, the nanocircuit impedance goes to infinity, corresponding to a voltage peak, while the current delivered by the source remains constant (assuming a non-zero resistive part of the impedance, that is, some loss). 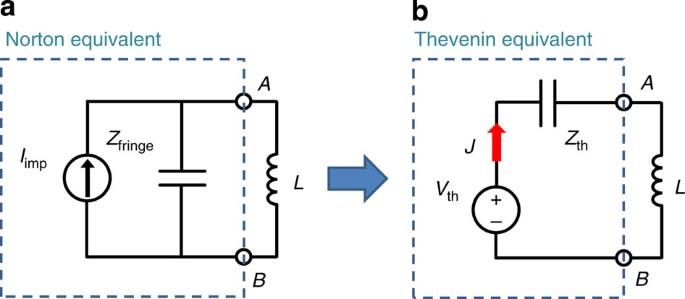Figure 6: Nanocircuit models. (a) Norton and (b) Thevenin equivalent nanocircuits for a subwavelength plasmonic nanoparticle excited by a uniform electric field. Two terminals A and B are defined on the upper and lower hemispherical surfaces of the particle and the circuit on the left (enclosed by the dashed box) can be equivalently represented in Norton or Thevenin form. Figure 6: Nanocircuit models. ( a ) Norton and ( b ) Thevenin equivalent nanocircuits for a subwavelength plasmonic nanoparticle excited by a uniform electric field. Two terminals A and B are defined on the upper and lower hemispherical surfaces of the particle and the circuit on the left (enclosed by the dashed box) can be equivalently represented in Norton or Thevenin form. Full size image In order to relate the circuit model to our measurements, we transform the original circuit in ref. 1 to its Thevenin equivalent ( Figs 2 and 6b ). At resonance, the current J delivered by the source is at maximum, directly related to the scattering peak observable in our experiments. From the physical standpoint, the current flowing in the circuit (red arrow in Figs 2c and 6b ) corresponds to the polarization currents sustaining the scattered fields. To better understand this issue, we define a pair of terminals A and B on the upper and lower hemispherical surfaces of the nanosphere, separating the impedance of the circuit element (the inductance L in this example) from the rest, as shown in Fig. 6a . The part on the left of the terminals, which includes the current source and the shunt fringe capacitance, can be substituted by its Thevenin equivalent circuit, composed of an equivalent voltage source V th in series with an equivalent impedance Z th ( Fig. 6b ). In particular, this equivalent voltage is the voltage obtained at the terminals AB when they are open-circuited. From ref. 1 , for a spherical particle of radius a and permittivity ε , the impressed current is I imp =− iω ( ε − ε 0 ) πa 2 | E 0 |, where E 0 is the incident electric field (assumed uniform), and the capacitive impedance associated to the fringe field is given above. The equivalent voltage source is therefore: where ε r = ε / ε 0 . The equivalent Thevenin impedance is the impedance at the terminals AB when the current source is open-circuited and, therefore, Z th = Z fringe . The final Thevenin equivalent circuit is shown in Fig. 6b , connected to the same nanoelement impedance, and consistent with Fig. 2 . This circuit, although equivalent from the point of view of the nanoelement, allows relating the scattering response to the current delivered by the voltage source. This quantity, in fact, is consistent with the polarization current induced in the nanocircuit, which is, in turn, directly related to the measured scattered field. In general, given a nanocircuit placed in an arbitrary environment, it is always possible to ‘pull out’ a pair of terminals and describe the surrounding space and sources with either a Norton equivalent (as in Fig. 6a ) or a Thevenin equivalent (as in Fig. 6b ). Thanks to the linearity of the electromagnetic problem, the two representations are equivalent from the point of view of the nanocircuit and, therefore, we can choose the circuit model better suited for our measurements. The introduction of this nanocircuit model is crucial to properly characterize the response of optical nanocircuits in the far-field. How to cite this article: Shi, J. et al. Modular assembly of optical nanocircuits. Nat. Commun. 5:3896 doi: 10.1038/ncomms4896 (2014).